Non-invasive mapping of deep-tissue lymph nodes in live animals using a multimodal PET/MRI nanoparticle The invasion status of tumour-draining lymph nodes (LNs) is a critical indicator of cancer stage and is important for treatment planning. Clinicians currently use planar scintigraphy and single-photon emission computed tomography (SPECT) with 99m Tc-radiocolloid to guide biopsy and resection of LNs. However, emerging multimodality approaches such as positron emission tomography combined with magnetic resonance imaging (PET/MRI) detect sites of disease with higher sensitivity and accuracy. Here we present a multimodal nanoparticle, 89 Zr-ferumoxytol, for the enhanced detection of LNs with PET/MRI. For genuine translational potential, we leverage a clinical iron oxide formulation, altered with minimal modification for radiolabelling. Axillary drainage in naive mice and from healthy and tumour-bearing prostates was investigated. We demonstrate that 89 Zr-ferumoxytol can be used for high-resolution tomographic studies of lymphatic drainage in preclinical disease models. This nanoparticle platform has significant translational potential to improve preoperative planning for nodal resection and tumour staging. The lymphatic system captures and transports extravasated material that escapes from connections between the arterial and venous systems. The lymphatics play a critical role to maintain homeostasis, while aberration in function often indicates the presence of disease [1] , [2] . Lymph node (LN) metastases are commonly the initial site of distant spread of cancer from a primary lesion, and invasion status of the LN surrounding a primary site is an important prognostic indicator of poor outcome [3] , [4] , [5] , [6] . Invasion status is therefore crucial information for disease stratification, staging and management. To acquire LN specimens for biopsy, current clinical practice involves the use of Isosulafan Blue dye and 99m Tc-radiocolloid. This two-step procedure utilizes the radiocolloid for sensitive localization of the sentinel, or first draining, node. The dye can then be used for intraoperative guidance by direct optical absorbance; however this requires full surgical exposure. This prevents any non-invasive LN imaging and precludes use in somatic locations, such as deep in the abdomen. 99m Tc-radiocolloid are nanoparticles composed of sulphur colloid or human serum albumin [7] , first employed over 50 years ago [8] . Used for whole body imaging for preoperative planning with planar lymphoscintigraphy or single-photon emission computed tomography (SPECT), they allow for subsequent intraoperative guidance by a handheld gamma-probe. Their widespread use makes this radiocolloid the most widely utilized nanomedicine for imaging [9] . Nanoparticle approaches are ideal to image the lymphatics as the size domain of such materials precludes either occlusion of micron-sized vessels or rapid diffusion into the blood and other compartments (as with small molecules) [10] . Numerous next-generation preclinical nanoparticles have demonstrated improvements over the low resolution and sensitivity of the single photon emitting 99m Tc colloid. A non-exhaustive list includes quantum dots [11] , metallic photoacoustic nanopaticles [12] , [13] , X-ray opaque bismuth sulphide particles [14] and liposomes for MR imaging [15] . Despite the great promise of this wide range of technologies for lymph imaging, there has been limited development of in-man use of next-generation nanoparticles for identifying tumour-draining LN since 1966. The most interesting translated work has used infrared dyes coupled to the colloid, either covalently (with IRDye800CW) [16] or non-covalently (with indocyanine green) [17] , or PET radiolabelling of the colloidal material [18] . Recently a new 99m Tc dextran preparation ‘Lymphoseek’ was approved for lymphosciintigraphy by the USFDA [19] . The greatest exception to the limited translation of recently developed contrast materials has been the use of iron oxide nanoparticles for systemic, rather than local, administration [20] . Iron oxide nanoparticles can be used in T 2 - or T 2 *-weighted MR imaging studies to produce contrast; the particles act as local magnetic inhomogeneities, decreasing signal at sites of their accumulation. However, the negative contrast generated by superparamagnetic iron oxide can be hard to interpret, and has realized limited adoption. For the imaging of local injection for draining LN, only isolated studies have been realized in the abdomen of healthy volunteers [21] or into the submucosa surrounding oesophageal masses [22] . We hypothesized that founding a multimodal particle upon the platform of an approved iron oxide particle formulation with an excellent toxicity profile (ferumoxytol [23] ) would enhance the diagnostic capacity of multimodal imaging in the clinical setting [24] , [25] . This approach takes advantage of the emerging positron emission tomography combined with magnetic resonance imaging (PET/MRI) platform to deliver high sensitivity and resolution, positive signal and quantitative information (from the PET imaging) while at the same time achieving high soft-tissue contrast by MRI [26] . Our results demonstrate high-sensitivity and high-resolution delineation of the nodes in axillary drainage models. In addition, the nanoparticle signal can be acquired by intraoperative detection devices as demonstrated in a genetically engineered mouse model of prostate cancer. The result is a multimodal next-generation nanoparticle for LN detection that has the potential to make the leap (back) to the clinic. Modification of ferumoxytol To prepare 89 Zr-radiolabelled iron oxide nanoparticles, it was necessary to modify the surface chemistry of the drug. 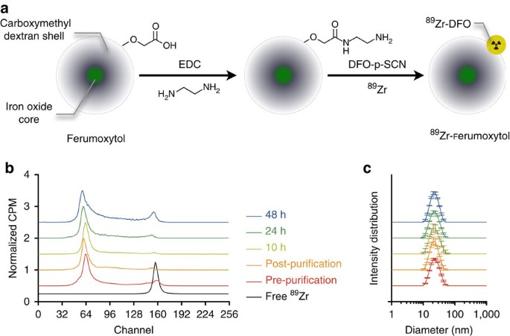Figure 1: Schematic of ferumoxytol radiolabelling and characterization. (a) Schematic of the carboxyl-terminated polyglucose sorbitol carboxymethylether coating (grey) surrounding the iron oxide crystal core (green) of the nanoparticle. Amination of the particles was carried out before their functionalization with ~7 DFO chelates. (b) Radiolabelling with89Zr was carried out in a high labelling efficiency reaction (>90%) before purification. Following gel filtration, the resulting PET-isotope functionalized ferumoxytol,89Zr-ferumoxytol, attained a >99% radiochemical purity, which was stable for over 24 h at 37 °C in mouse serum. Stacked plots of the radio-ITLC spectra are presented in normalized CPM, an arbitrary unit. (c) Particle size measurements before and following radiolabelling reveal no discernible change in diameter. Figure 1a summarizes the water-soluble carbodiimide chemistry employed to link the desferrioxamine chelate (DFO) to ferumoxytol to generate the PET/MRI contrast agent 89 Zr-DFO-labelled ferumoxytol ( 89 Zr-ferumoxytol). We used clinical samples of ferumoxytol, a US Food and Drug Administration approved agent for the treatment of iron deficiency by intravenous administration. The 17–35 nm nanoparticles are composed of an iron oxide core surrounded by a semisynthetic polysaccharide coating of polyglucose sorbitol carboxymethylether. With an R 2 relaxivity of 89 (mM s) −1 , these particles are potent T 2 - and T 2 *-weighted contrast agents [27] . Figure 1: Schematic of ferumoxytol radiolabelling and characterization. ( a ) Schematic of the carboxyl-terminated polyglucose sorbitol carboxymethylether coating (grey) surrounding the iron oxide crystal core (green) of the nanoparticle. Amination of the particles was carried out before their functionalization with ~7 DFO chelates. ( b ) Radiolabelling with 89 Zr was carried out in a high labelling efficiency reaction (>90%) before purification. Following gel filtration, the resulting PET-isotope functionalized ferumoxytol, 89 Zr-ferumoxytol, attained a >99% radiochemical purity, which was stable for over 24 h at 37 °C in mouse serum. Stacked plots of the radio-ITLC spectra are presented in normalized CPM, an arbitrary unit. ( c ) Particle size measurements before and following radiolabelling reveal no discernible change in diameter. Full size image We characterized the degree of chemical modification by determining the number of amine residues, DFO chelates and possible effects on particle size, relaxativity and charge. The reaction achieved amination of ~139±16 NH 2 ( n =5, ±s.d.) per particle, of which 7 were subsequently reacted with DFO. The particle diameter and relaxivity remained unchanged ( Supplementary Fig. 1 ). The addition of cationic charges to the surface of the particles only slightly altered the zeta potential from −17.6±1.36 to −16.43±0.85 mV ( n =5, ±s.d.). A large batch of amine-modified particles was used for subsequent experimentation. Overall, effects on particle size, charge and quantum properties were minimal. To assess the degree of radiolabelling and stability, we performed radio-instant thin layer chromatography (radio-ITLC; Fig. 1b , Supplementary Fig. 2 ). Chelated and conjugated activity does not move with the solvent front and remains at the spotting point (on the left as plotted). Over time, radiolysis and transmetallation contribute to some release of free 89 Zr-chelate complexes (that form peaks moving to the right, as plotted). Following a high radiolabelling efficiency (>90%), purification yielded 89 Zr-ferumoxytol with a specific activity of 0.28±0.08 mCi mg −1 Fe ( n =6 preparations). Greater specific activities can easily be achieved, however we chose a (low) value in the range of 0.1–0.5 mCi mg −1 Fe to achieve MR contrast on use with micro-dose PET imaging. Radiolabelling stability in serum at 37 °C provided encouraging results that the nanoparticles were stable when challenged. These are designed to break down and release iron over time, and by 48 h we had begun to see free 89 Zr migrating with the running buffer. No change in the diameter was observed under these conditions, confirming the stability of the radiolabeled particles ( Fig. 1c ). Axillary LN drainage To investigate the LN visualizing potential of 89 Zr-ferumoxtyol we first utilized a model of axillary lymph mapping by forepaw dermal injection [28] . Summarizing representative imaging results for PET/CT, MRI and PET/CT/MRI, the draining axillary and brachial nodes can be clearly detected tomographically at 6 h post-injection ( Fig. 2a–f ). By PET/CT, the two adjacent nodes (the brachial and axillary LN) atop the thoracic cage are seen with minimal background. 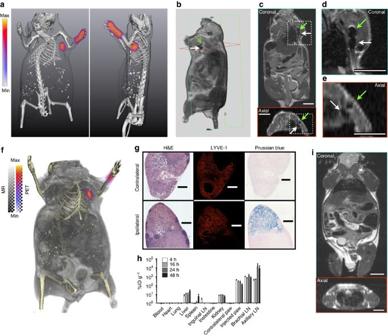Figure 2: Multimodal visualization of axillary lymph node group drainage. (a) 3D-rendered PET/CT imaging (two perspectives) of uptake in the brachial and axillary nodes. (b) 3D-rendered MRI (4.7 T) of the uptake in the two nodes. Hypointensity generated at the nodes (axillary, green arrow; brachial, white arrow) following uptake of the iron oxide nanoparticles can be clearly visualized in the volume rendering. (c) Coronal and axial planar images, as indicated from the boundary outlines on the 3D-rendered MR image. Here, we can clearly distinguish the draining axillary and brachial nodes from signal decrease (dark regions), in high-resolution. (d) Magnified images from the coronal and, (e) axial perspectives. (f) PET/CT/MR fusion of the nanoparticle distribution with detailed soft and hard tissues illustrates the advantage of preoperative planning for minimally invasive surgery. The method used for co-registration of these three image sets (independently acquired) is detailed in Methods. (g) Histological verification of the lymphotropic clearance of tracer. Dense follicular staining by haematoxylin and eosin (H&E) and LYVE-1 positive immunofluorescent staining are concordant with the presence of nanoparticles draining from the injection site. No Prussian blue (PB) development of iron oxide is found in the contralateral nodes. Micrograph scale bars are 500 μm in length. (h) Localization of the particles to the LN draining the injection site is specific, rapid and sustained over time (n=5 animals per time point; ±s.e.m.). Nanoparticles filtered through the lymphatics re-enter the vasculature and take residence in the liver. As the biocompatible particles break down to release their iron payload, the small molecule89Zr-DFO is cleared by renal filtration. (i) In the absence of89Zr-ferumoxytol PET or MR contrast, the submillimeter (diameter) LN are exceptionally difficult to discern, even at higher MR resolution than the scans used in this work. All scale bars for MR images are 0.8 cm. Figure 2: Multimodal visualization of axillary lymph node group drainage. ( a ) 3D-rendered PET/CT imaging (two perspectives) of uptake in the brachial and axillary nodes. ( b ) 3D-rendered MRI (4.7 T) of the uptake in the two nodes. Hypointensity generated at the nodes (axillary, green arrow; brachial, white arrow) following uptake of the iron oxide nanoparticles can be clearly visualized in the volume rendering. ( c ) Coronal and axial planar images, as indicated from the boundary outlines on the 3D-rendered MR image. Here, we can clearly distinguish the draining axillary and brachial nodes from signal decrease (dark regions), in high-resolution. ( d ) Magnified images from the coronal and, ( e ) axial perspectives. ( f ) PET/CT/MR fusion of the nanoparticle distribution with detailed soft and hard tissues illustrates the advantage of preoperative planning for minimally invasive surgery. The method used for co-registration of these three image sets (independently acquired) is detailed in Methods. ( g ) Histological verification of the lymphotropic clearance of tracer. Dense follicular staining by haematoxylin and eosin (H&E) and LYVE-1 positive immunofluorescent staining are concordant with the presence of nanoparticles draining from the injection site. No Prussian blue (PB) development of iron oxide is found in the contralateral nodes. Micrograph scale bars are 500 μm in length. ( h ) Localization of the particles to the LN draining the injection site is specific, rapid and sustained over time ( n =5 animals per time point; ±s.e.m.). Nanoparticles filtered through the lymphatics re-enter the vasculature and take residence in the liver. As the biocompatible particles break down to release their iron payload, the small molecule 89 Zr-DFO is cleared by renal filtration. ( i ) In the absence of 89 Zr-ferumoxytol PET or MR contrast, the submillimeter (diameter) LN are exceptionally difficult to discern, even at higher MR resolution than the scans used in this work. All scale bars for MR images are 0.8 cm. Full size image Superparamagnetic nanoparticles cause local inhomogeneities in the magnetic field, causing decoherence of protons’ precession. This results in negative or ‘dark’ contrast in the LN by MR imaging. Magnified images of the relevant area clearly show the presence of particle contrast in the LN. Images were fused using a PET/CT and MRI/CT technique [29] , enabling trimodality PET/CT/MRI fusion. This illustrates the value of multimodality imaging for presurgical planning. Here, we can locate the draining nodes contextualized deep in their soft-tissue milieu ( Fig. 2f ). Histological examination recapitulates the imaging results for LN specific staining and the presence of iron solely in the nodes draining from the injection site ( Fig. 2g ). The acute biodistribution of 89 Zr-ferumoxtyol confirms the lymphatic drainage from the dermal injection model ( Fig. 2h and Supplementary Fig. 3 ). Particles clear from the injection site and reside at the node. Some uptake seen at the earliest time point of 4 h is seen in nodes not draining from the injection site, a combination of some of the injectate accessing the blood stream and free 89 Zr-DFO from the biodegradable particles. Comparison by MR imaging alone (without the PET or T 2 *-weighted iron oxide signal) demonstrates the difficulty in detection of these submillimeter structures without contrast ( Fig. 2i and Supplementary Fig. 4 ). These results are in contrast to the results of imaging the same draining LN in the mouse using the conventional 99m Tc-radiocolloid and SPECT/CT imaging ( Supplementary Figs 5 and 6 ). The modality presents a significantly higher background, even after imaging acquisition times fourfold longer than the PET/CT approach. The images using SPECT and PET were acquired at the same time post-injection (6 h); however, detection of the draining nodes was possible as early as 1 h post-injection with 89 Zr-ferumoxytol. Prostatic drainage Using a sliding laparoscopy inoculation procedure, ~5 μl of 89 Zr-ferumoxytol was administered to the right anterior prostate (AP). PET/CT imaging 6 h following administration reveals the site of the injection and clearly delineates three draining LN ( Fig. 3a ). MRI provides the complementary anatomic topography of the abdomen, with signal decrease at the draining LN ( Fig. 3b ). An enlarged abdominal area in Fig. 3c provides clearer detection of the two in-plane nodes by MRI, which drain from the AP injection (a schematic diagram of the prostate is provided for reference, Fig. 3d ). 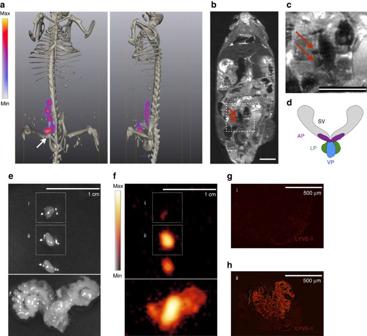Figure 3: Intraprostatic administration reveals pelvic lymph node distribution for therapy planning and surgical confirmation. 89Zr-ferumoxytol (5 μl, 35 μCi) was administered to the AP. Imaging was conducted ~6 h after injection. (a) PET signal is present at the site of the injection (arrow and asterisk) and at three somatic nodal stations draining from the AP as visualized by PET/CT. (b) The negative contrast produced by the nanoparticles is visible in a whole body coronal MR slice (red arrows). (c) On greater magnification of the coronal MR image, it is possible to distinguish two in-plane draining nodes from signal voids created by the nanoparticles (red arrows), however this task is difficult with MRI alone as there are other regions of low signal intensity. Scale bars on MR images are 0.8 cm. (d) For reference to the following dissection, a schematic diagram of the mouse prostate organ is provided showing the SV, seminal vesicles; LP, lateral prostate; VP, ventral prostate and AP, anterior prostate. (e) PET and MRI were used as preoperative planning tools for radical prostatectomy and LN dissection, by visual guidance. A white light macrograph of the excised tissues with 1 cm scale is shown. (f) In order to verify that the targeted structures were indeed removed,ex vivoPET was performed. Intraoperatively, this role could be carried out with a handheld beta probe. The AP and two of the excised specimens were detected by PET. (g) The signal free specimen (i) was negative for LYVE-1 staining for lymphatic endothelium. (h) However, the radioactive tissue (ii) was indeed confirmed to be a LN; scale bars for micrographs are both 500 μm. This indicates that89Zr-ferumoxytol provides the potential for intraoperative real-time confirmation of the surgical resection of sites of interest. Figure 3: Intraprostatic administration reveals pelvic lymph node distribution for therapy planning and surgical confirmation. 89 Zr-ferumoxytol (5 μl, 35 μCi) was administered to the AP. Imaging was conducted ~6 h after injection. ( a ) PET signal is present at the site of the injection (arrow and asterisk) and at three somatic nodal stations draining from the AP as visualized by PET/CT. ( b ) The negative contrast produced by the nanoparticles is visible in a whole body coronal MR slice (red arrows). ( c ) On greater magnification of the coronal MR image, it is possible to distinguish two in-plane draining nodes from signal voids created by the nanoparticles (red arrows), however this task is difficult with MRI alone as there are other regions of low signal intensity. Scale bars on MR images are 0.8 cm. ( d ) For reference to the following dissection, a schematic diagram of the mouse prostate organ is provided showing the SV, seminal vesicles; LP, lateral prostate; VP, ventral prostate and AP, anterior prostate. ( e ) PET and MRI were used as preoperative planning tools for radical prostatectomy and LN dissection, by visual guidance. A white light macrograph of the excised tissues with 1 cm scale is shown. ( f ) In order to verify that the targeted structures were indeed removed, ex vivo PET was performed. Intraoperatively, this role could be carried out with a handheld beta probe. The AP and two of the excised specimens were detected by PET. ( g ) The signal free specimen (i) was negative for LYVE-1 staining for lymphatic endothelium. ( h ) However, the radioactive tissue (ii) was indeed confirmed to be a LN; scale bars for micrographs are both 500 μm. This indicates that 89 Zr-ferumoxytol provides the potential for intraoperative real-time confirmation of the surgical resection of sites of interest. Full size image This functional and anatomic imaging was used to plan surgical resection of the four positive sites. The surgeon, then operating solely by eye, ostensibly excised the prostate and the three LN ( Fig. 3e ). However, ex vivo PET of the tissues revealed that while the AP and two of the tissues presented high signal, the third structure did not ( Fig. 3f ). Subsequent investigation confirmed that the tissue without signal was negative for markers of the lymphatic endothelium ( Fig. 3g,h ), and thus the surgeon had not resected the final draining node. In the clinical setting, a gamma probe, Cerenkov camera or other radiation detection device could easily be used to detect 89 Zr-ferumoxytol to determine successful surgery. Drainage in a genetically engineered mouse model of prostate cancer The normal mouse organ is several millimetres in diameter, while the hypertrophic tumorous prostate of the Hi-Myc mouse is considerably enlarged ( Fig. 4a–c ). Following intraprostatic administration of 89 Zr-ferumoxytol into diseased mice, PET/MR imaging is able to reveal the lymphatic distribution from the AP. 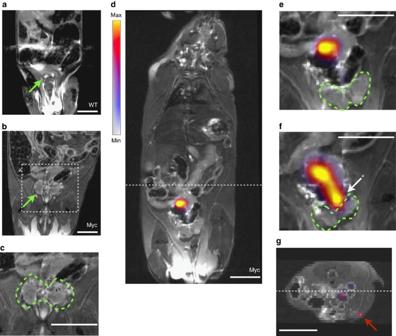Figure 4: Determining local and extended lymphatic transport in a transgenic model of prostate cancer. (a) Coronal MR T2-weighted image of a representative healthy wild-type C57BL/6 mouse (WT). Whole body images are shown inSupplementary Fig. 7. Green arrow indicates the ventral prostate (VP), as the smaller AP cannot be easily seen in living mice. (b) MRI under the same imaging conditions of an age matched Hi-Myc mouse, which expresses human c-Myc in the mouse prostate (Myc). The hypertrophic prostate can be easily distinguished (green arrow). (c) Magnification of the area defined from the previous image, with the tumorous prostate outlined. (d) Whole body PET/MRI fused slice of89Zr-ferumoxytol in a draining LN, 6 h post-injection. (e) Magnified prostate region distinctly shows that the draining LN is outside of the prostate organ. The VP in this slice is delineated by a dashed green outline. (f) In the preceding coronal slice, the site of injection in the AP (arrow and asterisk) can be seen along with the draining lymphatic channel. (g) In the reconstructed axial orientation (located at the hashed marks on the coronal image), sensitive PET detection enables visualization of tracer in a more distant draining inguinal node (red arrow). In the clinical context, the detection of a draining LN outside of the pelvic bed would necessitate a widened field of biopsy sampling or therapeutic intervention. All scale bars are 0.8 cm in length. Figure 4d provides a representative coronal whole body PET/MRI example of the tracer uptake at a draining node, 6 h following injection. Figure 4: Determining local and extended lymphatic transport in a transgenic model of prostate cancer. ( a ) Coronal MR T 2 -weighted image of a representative healthy wild-type C57BL/6 mouse (WT). Whole body images are shown in Supplementary Fig. 7 . Green arrow indicates the ventral prostate (VP), as the smaller AP cannot be easily seen in living mice. ( b ) MRI under the same imaging conditions of an age matched Hi-Myc mouse, which expresses human c-Myc in the mouse prostate (Myc). The hypertrophic prostate can be easily distinguished (green arrow). ( c ) Magnification of the area defined from the previous image, with the tumorous prostate outlined. ( d ) Whole body PET/MRI fused slice of 89 Zr-ferumoxytol in a draining LN, 6 h post-injection. ( e ) Magnified prostate region distinctly shows that the draining LN is outside of the prostate organ. The VP in this slice is delineated by a dashed green outline. ( f ) In the preceding coronal slice, the site of injection in the AP (arrow and asterisk) can be seen along with the draining lymphatic channel. ( g ) In the reconstructed axial orientation (located at the hashed marks on the coronal image), sensitive PET detection enables visualization of tracer in a more distant draining inguinal node (red arrow). In the clinical context, the detection of a draining LN outside of the pelvic bed would necessitate a widened field of biopsy sampling or therapeutic intervention. All scale bars are 0.8 cm in length. Full size image Magnification of the relevant prostatic area distinctly shows the draining LN rostral exterior to the prostate ( Fig. 4e ). In the preceding slice, again enlarged, we can discern the AP injection site and a draining lymphatic channel leading to the draining LN ( Fig. 4f , whole body images are presented in Supplementary Fig. 7 ). In addition, we are able to identify LN uptake of the particles outside of the pelvis, notably inguinal nodes, a representative figure is shown in the axial orientation ( Fig. 4g ). Such a finding in a patient would alter surgical and therapeutic management of the disease. Nanoparticle development and application is an area of intense research in the biomedical field. Unique physical and chemical properties emerge at the nanometre dimension, and this is the length scale over which living systems interact with their surroundings. Despite the sheer number of nanoparticle imaging and therapeutic agents produced to date, very few have been evaluated in humans, let alone approved for conventional use. This work was motivated by the goal of multimodal mapping of the lymphatics in small animals using a mildly-derivatized clinically approved compound in microdose amounts. Ferumoxytol is an approved iron replacement nanoformulation that has also been used as an MR contrast-enhancing agent. At this time, there are a total of 42 trials that are actively recruiting or have been completed with this agent on the registry database ClinicalTrials.gov. The chemical modifications made in this work enable local administration for PET imaging of this MR contrast agent. While such changes are subject to review by supervisory medical regulatory agencies, our characterization revealed that such changes to the particles did not significantly affect the surface charge, size or relaxivity. Previously, imaging of the lymphatic system in the clinic has relied primarily on local administration of 99m Tc-colloids and isosulfan blue. A recent development has been the combination of the colloid with the clinically approved indocyanine green fluorophore. This approach allows for multimodal SPECT and fluorescence guided resection of draining LNs in both pre- and clinical settings [30] , [31] . In a related strategy, others have covalently modified the albumin colloid with 89 Zr-DFO (rather than with 99m Tc) for preclinical drainage mapping in rabbits [32] and man [18] , as well as with IRDye800CW for multimodal imaging [33] . Further developments in the radio- and radio-fluorescence guidance are expected in the near future. While an area of intense interest, emerging PET/MRI bimodality scanners possess several distinct advantages over the current paradigm of PET/CT and SPECT/CT systems. Most prominently, the greatly enhanced soft-tissue contrast of magnetic resonance imaging is able to localize PET contrast agents with greater anatomical information. In the context of nanoparticulate contrast for LN distinction, the use of PET versus SPECT technology in the clinic results in higher sensitivity (with the added benefit of reduced dose), greater resolution and critically reduced partial volume effects. The CT radiation dose is also removed. Our work has shown that PET/MRI can be used to localize the draining lymphatics in healthy mice in both the axillary and the abdominal regions. Drainage to the brachial and axillary nodes was visualized by defined hypointense contrast on MRI as well as localized annihilation-photon signal on PET. The nodes could be detected as early as 1 h after injection of the tracer, and were sustained for the 6 h imaging time points presented here. As ferumoxytol is designed for degradation and iron release in vivo , purification of the 89 Zr-ferumoxytol immediately before use is required to minimize background signal. SPECT studies of 99m Tc-SC uptake were also able to distinguish the draining node. However, greater activity and longer scan times were required. Mapping of the peripheral LN architecture above can be accomplished by other approaches at shallow tissue depths (for example, fluorescent particles) in regions such as the axilla. However, visualization of the nodal drainage in deeper tissues is generally not possible with these techniques without first performing surgical exposition. This technique, demonstrated first with 99m Tc-colloid, to directly inject into an organ or around a tumour, is emerging as a powerful tool to better plan surgical intervention or to determine the boundaries of therapeutic radiation fields [17] , [34] , [35] , [36] . Therefore, we assessed the ability of 89 Zr-ferumoxytol to interrogate the deep somatic lymphatics of the pelvis following intraprostatic injection of the tracer. In the abdomen, the combined utility of PET/MRI demonstrates the ability of 89 Zr-ferumoxytol to map the draining lymphatics from the prostate with the soft-tissue context of the surrounding organs. Pre-, intra- and postoperative guidance are important steps in the later-stage therapeutic decision process. Greater understanding of disease, in this example prostate cancer, and its spread through the lymphatics have been stymied in part because non-invasive deep tissue imaging of small animal models is so difficult. Previous work with iron oxides have highlighted that the negative contrast generated by these nanoparticles can be difficult to interpret. In the abdomen, there are many other structures and voids that also present as low signal regions. With the additional PET signal, identification of the nodes can be made rapidly. 89 Zr-Ferumoxtyol could be a critically important tool providing additional insight into lymphatic function in non-invasively imaging disease models. To test this hypothesis we evaluated the distribution of nanoparticles in Hi-Myc transgenic mice. Hi-Myc mice exhibit invasive adenocarcinoma of the prostate between 6 and 9 months, which bears features similar to human disease. On direct administration to the prostate, we were able to delineate draining nodes in the abdomen by PET. As well, uptake in inguinal nodes further from the prostate was visualized using fused PET/MRI. This high-resolution and high-sensitivity has potentially important implications for enhanced study of the lymphatic drainage in murine models of disease. The detection of lymph drainage from the prostate to a specific site, such as the inguinal node, has important ramifications in the context of guiding biopsy, surgical excision following radical prostatectomy, or external beam radiation therapy planning. These results demonstrate the value for a new, high resolution, multimodal tool for preclinical imaging of the lymphatic system. We assessed deep-tissue lymphatic function and drainage using PET/MRI, widening the degree to which investigators may examine the effects of tumours on the lymphatic system. In addition, in the clinical setting the ability to sensitively detect local drainage outside of the pelvic bed would motivate additional biopsy and/or therapeutic contingencies. The ability of 89 Zr-ferumoxytol to provide information-rich preoperative mapping as well as intraoperative confirmation augment its capacity to evaluate preclinical disease models. The rapid degradation of the compound in vivo necessitates purification before use. However, we expect that the described radiolabeled nanoparticle platform will have widespread use in diverse nanomedical diagnostic applications, extending the successful use of nanoparticles for imaging ( 99m Tc-radiocolloid) in the clinic. Materials All reagents were supplied by ThermoFisher Scientific, unless otherwise noted. 89 Zr-ferumoxytol Ferumoxytol (AMAG Pharmaceuticals) was buffer exchanged by PD-10 Column (GE Healthcare) into (2-( N -morpholino) ethanesulfonic acid) MES buffer (0.5 M, pH 5). To 14 mg of elemental iron (90 μM nanoparticles) was added 25 mg of 1-Ethyl-3-(3-dimethylaminopropyl) carbodiimide. The sample was mixed for 5 min in a dry bath at 25 °C. Ethylenediamine (100 μl) was added followed by 1 N hydrochloric acid to adjust to pH 6. The reaction continued, mixing at room temperature for 2 h. Nanoparticles were purified on PD-10 equilibrated with phosphate buffered saline (PBS), followed by serial purification and concentration on Amicon Ultra 50 kDa MWCO (Millipore) into PBS, pH 7.4. Desferrioxamine conjugation using DFO-p-SCN (Macrocyclics) was performed in pH 8, 0.1 M 4-(2-hydroxyethyl)-1-piperazineethanesulfonic acid (HEPES) buffer at a molar ratio of 15:1 per particle. Particle concentration was assessed by utilizing a spectrophotometric iron digestion assay [37] . The reaction was purified by PD-10 and subsequently concentrated by Amicon Ultra 50 kDa filtration. Zirconium-89 was produced via the 89 Y( p , n ) 89 Zr transmutation reaction on an EBCO TR19/9 variable-beam energy cyclotron (Ebco Industries). The [ 89 Zr]Zr-oxalate was isolated in high radionuclidic and radiochemical purity >99.99%. [ 89 Zr]Zr-oxalate was balanced to pH 7.2 using sodium carbonate, as described [38] . [ 89 Zr] was added to the chelate modified ferumoxytol and mixed at 37 °C for 1 h. The sample was then spin filtered using a 50 kDa filter (YM50; Amicon) until pure, and reconstituted to the starting volume in saline. Probe characterization The number of amines conjugated per particle was assessed by reaction with N -Succinimidyl 3-(2-pyridyldithio)-propionate and subsequent cleavage with Tris (2-carboxyethyl) phosphine hydrochloride. Spectrophotometric measurement and quantification was made, as described, with purification by PD-10 rather than precipitation [37] . Particle size and zeta potential measurements were made on the original and modified particles by dynamic light scattering (Malvern NanoZS). The number of DFO per particle was determined by the number of amine residues consumed, as above. Relaxivity of the particles was measured using a tabletop relaxometer (Bruker Minispec; 20 MHz at 40 °C). Radiolabelling purity was assessed by radio-ITLC (Bioscan System 200 Imaging Scanner), using the Win-Scan Radio-TLC software (version 2.2) and 89 Zr-radiolabelling reactions were monitored by using silica-gel impregnated glass-fibre TLC paper (Pall Corp.). Running solvent was 50 mM ethylenediaminetetraacetic acid (pH 5.5). Radiostability tests were performed with repeated radio-ITLC measurements of the 89 Zr-ferumoxytol incubated in murine serum at 37 °C over 48 h. At the same time points, nanoparticle size measurements were made by dynamic light scattering. Small-animal experiments Animal experiments were in accordance with guidelines from the Institutional Animal Care and Use Committee and with the Guide for the Care and Use of Laboratory Animals from the National Institutes of Health (NIH). All animal procedures were performed under anaesthesia by inhalation of a 1–2% iso-flurane–air mixture (Baxter Healthcare). Animals were obtained from either Harlan Laboratories and/or maintained in-house at MSKCC (Hi-Myc mice). Female C57BL/6 mice were used for axillary LN imaging and biodistribution (~8 weeks of age). For intraprostatic injection studies, male C57BL/6 and Hi-Myc mice were age matched (35–46 weeks of age) before experimentation for imaging. Surgical procedures were performed using sterilized instruments in a laminar flow hood. Animals were anesthetized by means of isofluran inhalation (1.5–2%), and ophthalmic ointment was applied. Animals were placed in a supine position, under a sterile drape. The mouse abdomen was shaved before sterilization with triplicate topical application of povidone-iodine and ethanol. A midline incision was made in the lower abdomen, ~10 mm in length, using a disposable scalpel (all equipment Fisher Scientific, unless otherwise noted). The seminal vesicles were lifted to expose the prostate tissue with curved dissecting forceps. The nanoparticle formulation was slowly inoculated into the right AP using a hypodermic needle (30-gauge × 1.9 cm (0.75 in), Kendall Monoject; Tyco Healthcare). The needle was left in the tissue for ~20–30 s after the injection, to prevent spilling of contrast back into the abdominal cavity. Correct inoculation could be immediately assessed, as visual assessment of any leakage can easily be detected from the injection site due to the dark colour of the solution. Animal imaging Imaging was performed on the following instruments using a custom-built restraint device for registered PET, CT and MR image data [29] . Briefly, anesthetized mice were placed on a non-magnetic polymethylmethacrylate bed. The animal was placed at a fixed position relative to the animal bed using thin 0.01-mm polyethylene wrapping, which accommodates a nose cone for the continued administration of oxygen and gaseous anaesthesia. The restraint provided by the wrap effectively restricts the movement and has the added advantage of applying a light pressure over the entire body of the animal to reduce respiratory artefacts. Registration between the modalities is then dependent on establishing a frame of reference relative to the bed for each scanner and calculating the rigid transforms between them. In addition, to MR and CT data were co-registered using the rigid (6 degrees of freedom) optimized automatic least squares three-dimensional registration algorithm of surfaces of the Medical Image Processing, Analysis and Visualization software from the Center for Information Technology at NIH [39] . PET image data were corrected for detector non-uniformity, dead time, random coincidences and physical decay. PET images were acquired on the Focus 120 microPET small-animal scanner (Concorde Microsystems Inc.) with an energy window of 350–700 keV and coincidence-timing window of 6 ns. PET data were reconstructed using a maximum a priori MAP and 3D filtered back projection and reconstruction using a ramp filter with a cut-off frequency equal to the Nyquist frequency into a 128 × 128 × 95 matrix [40] . The minimal volume of 89 Zr-DFO-ferumoxytol that was possible to repeatedly administer was injected, ~4–6 μl. This resulted in an approximate activity dose of 1.3 MBq and an elemental iron dose of ~0.25 mg. CT imaging was conducted on the Bioscan NanoSPECT/CT with 55 kVp, a pitch of 1 with 240 projections in a spiral scan mode. The entire animal was scanned using a multiple field of view procedure (with an approximate field of view of 4 × 4 × 6 cm per bed position), commonly requiring three bed positions per scan. Total scan time was ~12 min. A Shepp-Logan filter was used during the reconstruction process to produce image matrices with isotropic volumes of 221 μm. MR imaging was performed on a Bruker BioSpin 4.7 T. A whole body coronal T 2 -weighted turbo spin echo sequence (3,200/57.1) with 8 averages was used, with slice dimensions of 8.5 × 3.99 × 0.8 cm. Total scan duration was 10 min 14 s. Scale of the images are 220 μm per pixel in plane and 800 μm out of plane. An original DICOM image is presented as Supplementary Fig. 8 . Ex vivo PET was performed by placing excised tissue in a 50 mm polystyrene tissue culture dish with a coating of ice-cold PBS. Samples were scanned for ~8 min. The ex vivo PET acquisition was reconstructed using a filtered back projection algorithm. A minimum of at least four mice were imaged for each experimental model. SPECT/CT imaging Approximately 5.5 MBq of 99m Tc-sulphur colloid was injected into the right mouse forepaw (~12 μl). The particles were given 6–8 h to accumulate in the draining node and subsequently imaged using the NanoSPECT (Bioscan), which possesses four 215 × 230 mm 2 NaI crystals and 33 PMT elements. SPECT images were acquired using an energy window around the 140.95 keV peak (window width of 14 keV) for ~50 min with 20 projections using the highest-sensitivity 2 mm pinhole collimators (nine holes per head). The field of view on the nanoSPECT is extended using a step-and-shoot helical scan of the animal, with the user defining a range from 24 to 270 mm according to the region to be imaged. Here, an axial field of view of 38 mm was set, and the length of the animal was scanned. Reconstruction was performed using a 256 × 256 in-plane matrix using the HiSPECT software (Scivis GmbH). Co-registered CT images were acquired at 55 kVp. SPECT and CT images were reconstructed, fused and analysed with InVivoScope (Bioscan). Molecular imaging visualization Data visualization was accomplished with a combination of the open source FIJI (NIH) [41] , ASIPro (Concorde Microsystems) and Amira 5.3.3 (FEI). FIJI was used to generate whole body 3D images of the MR acquisitions. Fused and nuclear medicine tomographic images were generated using Amira. These images are 3D volume rendering of PET or SPECT data overlaid onto surface-rendered CT data (or CT and MR data). To generate these images, a weighted average of the intensities along projections through the PET is computed and this in turn is blended with the CT-rendered image. The three dimensionally rendered MR data used an alpha transfer function (mapping transparency to intensity) included as Supplementary Fig. 9 . To show the PET data are represented with a semiquantitative blue (low)–yellow (high) colour scale; the SPECT data uses a green (low)–blue (high) colour scale. Immunofluorescence and immunohistochemistry Excised tissues were embedded in optimal cutting temperature compound (OCT; TissueTek), frozen and sectioned at 8 μm using a cryotome (−18 °C; HM 500 M cryostat, Microm). Serial sections were stained using haematoxylin and eosin, incubated with LYVE-1 (AF413 mouse monoclonal diluted at 1:1,000; R&D Systems) or developed for iron oxide (Prussian Blue stain kit). For LYVE-1 immunofluorescence secondary staining, Alexa Fluor 594 was used (Life Technologies). All microscopy was performed on an EclipseTi using the Elements software package (Nikon). A LYVE-1-stained micrograph of the slide containing slices of all three of the resected tissues from the surgical-confirmation experiment are presented in Supplementary Fig. 10 . Biodistribution Animals were injected dermally on the back of the forepaw with ~25 μCi (0.925 MBq) in ~10 μl. At serial time points, animals ( n =5) were euthanized by CO 2 (gas) asphyxiation. Major organs, the site of injection, the contralateral limb and LNs were dissected from the killed mice. Background-corrected count-per-minute data of the excised tissues were acquired on an automatic Wizard γ-counter (Perkin Elmer) using an energy window of 800–1,000 keV for 89 Zr (909 keV emission). Statistical analyses Data were analysed by using the unpaired, two-tailed Student’s t -test. Differences at the 95% confidence level ( P <0.05) were considered to be statistically significant. How to cite this article: Thorek, D. L. J. et al . Non-invasive mapping of deep-tissue lymph nodes in live animals using a multimodal PET/MRI nanoparticle. Nat. Commun. 5:3097 doi: 10.1038/ncomms4097 (2014).